Revisiting the role of histo-blood group antigens in rotavirus host-cell invasion Histo-blood group antigens (HBGAs) have been proposed as rotavirus receptors. H type-1 and Lewis b antigens have been reported to bind VP8* from major human rotavirus genotypes P[4], P[6] and P[8], while VP8* from a rarer P[14] rotavirus recognizes A-type HBGAs. However, the role and significance of HBGA receptors in rotavirus pathogenesis remains uncertain. Here we report that P[14] rotavirus HAL1166 and the related P[9] human rotavirus K8 bind to A-type HBGAs, although neither virus engages the HBGA-specific α1,2-linked fucose moiety. Notably, human rotaviruses DS-1 (P[4]) and RV-3 (P[6]) also use A-type HBGAs for infection, with fucose involvement. However, human P[8] rotavirus Wa does not recognize A-type HBGAs. Furthermore, the common human rotaviruses that we have investigated do not use Lewis b and H type-1 antigens. Our results indicate that A-type HBGAs are receptors for human rotaviruses, although rotavirus strains vary in their ability to recognize these antigens. Rotaviruses, members of the Reoviridae family, are the most important cause of severe diarrhoeal disease and dehydration in young children with around 500,000 deaths each year [1] . The introduction of two vaccines licensed in 2006 and 2008 has been successful in reducing disease severity and death rates [2] . However, several recent studies have revealed a significant increase in intussusception after the administration of the first or second rotavirus vaccine dose [3] , [4] , and vaccine-associated hospitalizations for severe rotavirus gastroenteritis have been reported [5] . These risks must be weighed up against the benefits of preventing rotavirus-associated illness. Rotaviruses with the P[8] genotype of the spike protein VP4 are predominantly associated with severe disease globally, with the P[4] and P[6] genotypes being substantially less common [6] . Virus infectivity is activated by trypsin cleavage of VP4 to produce the VP5* and VP8* subunits. Although both subunits remain associated on the virion surface, initial cell attachment to host cell membrane glycoconjugates is mediated by the VP8* head of the spike protein [7] , [8] . Gangliosides are glycosphingolipids with one or more sialic acid residues that are key receptor molecules for rotavirus infection [9] , [10] , [11] , [12] , [13] , [14] . Rotaviruses have been classified as sialidase-sensitive or sialidase-insensitive, based on the effect on their infectivity of host cell pre-treatment with sialidase. However, commonly used bacterial and viral sialidases remove only terminal sialic acids from sialylglycoconjugates. Sialic acid recognition by sialidase-sensitive animal rotaviruses via VP8* is structurally well characterized through a series of crystallographic studies [13] , [15] , [16] , [17] , [18] , [19] , [20] , [21] . Our recent studies using nuclear magnetic resonance (NMR) spectroscopy and cell-based assays identified GM1 as a ganglioside receptor for the human rotavirus strains Wa (P[8]) and RV-3 (P[6]), and revealed that the internal N -acetylneuraminic acid (sialic acid) residue of GM1 plays a key role in VP8* recognition [12] , [22] . We concluded that human sialidase-insensitive strains such as Wa and RV-3, and most probably other human strains, require the presence of sialic acid-containing receptors for efficient infection [12] , [22] . A new paradigm of human P[14] rotavirus binding to A-type HBGA has been recently suggested, related to decreased infectivity of HAL1166 in HT-29 cells following anti-A-type antibody treatment and increased infectivity in CHO cells expressing A-type HBGA (ref. 23 ). The X-ray crystal structure of HAL1166 VP8* revealed a typical galectin-like fold with the twisted β-sheets separated by a shallow cleft as observed in all available VP8* structures, including those of the sialidase-insensitive human rotaviruses Wa and DS-1 (P[4]), and the sialidase-sensitive animal strains RRV and CRW-8 VP8* (refs 16 , 23 ). Notably, the width of the binding site in HAL1166 VP8* appears narrower than in Wa and DS-1, resembling the binding site of RRV and CRW-8. Interestingly, sialic acids bind the VP8* of such animal rotaviruses at the same location within the narrow cleft as HBGA A-type trisaccharide (A-tri) and tetrasaccharide (A-tetra) binds to HAL1166 VP8*, although the key amino acids that interact with sialic acids and HBGA are different. Based on VP8* sequence alignments and rotavirus infectivity assays, it was predicted that the human P[9] rotavirus K8 could also bind to A-type HBGA, although no structural evidence has been reported. The VP8* of P[9], P[14] and P[25] genotype rotaviruses within P genogroup III bind A-type HBGAs in haemagglutination inhibition and synthetic oligosaccharide-based assays [24] . In addition, binding assays with P genogroup II rotaviruses of P genotypes [4], [6] and [8] showed interaction of H type-1 and Lewis b antigens with the VP8* of P[4] and P[8] human rotaviruses, while P[6] rotavirus VP8* bound only to H type-1 antigen [25] , [26] . In the current study, we sought to determine the importance of HBGA receptors for several major human rotavirus genotypes. Our results demonstrate that A-type HBGAs are important receptors for human rotaviruses, although major variations between virus strains were detected. Using a multidisciplinary approach, we show that P[14] rotavirus HAL1166 and the related P[9] human rotavirus K8 bind A-type HBGAs without engaging the HBGA-specific α1,2-linked fucose moiety. Importantly, human rotaviruses DS-1 (P[4]) and RV-3 (P[6]) also use A-type HBGAs for infection, with fucose involvement. In contrast, the human P[8] rotavirus Wa does not recognize A-type HBGAs and no rotavirus strain we tested uses H-type-1 and Lewis b antigens. Binding of HBGAs to rotavirus VP8* The evidence supporting the notion that HBGAs are common cell receptors for human rotaviruses remains incomplete and unclear. To address this issue, we report here an NMR solution study of the interactions between A-tri and A-tetra ( Fig. 1a ), and the VP8* carbohydrate-recognizing domain from human rotaviruses HAL1166 (P[14, III]), K8 (P[9, III]), Wa (P[8, II]), RV-3 (P[6, II]) and DS-1 (P[4, II]). The 1 H NMR spectrum of A-tri under our experimental conditions ( Fig. 1b ) revealed existence of α- and β-pyranose (six-membered ring) and -furanose (five-membered ring) forms in aqueous solution that are populated as follows ( Fig. 1c ): 52% GalNAcα1,3[Fucα1,2]Gal p α (A-tri p α ), 24% GalNAcα1,3[Fucα1,2]Gal p β (A-tri p β ), 18% GalNAcα1,3[Fucα1,2]Gal f α(A-tri f α ) and 6% GalNAcα1,3[Fucα1,2]Gal f β (A-tri f β ), consistent with a previous report [27] . 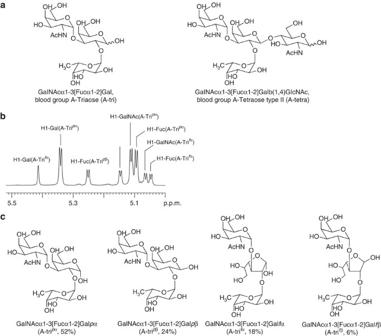Figure 1: Structures and NMR spectra of A-tri and A-tetra glycans. Structures of A-type HBGAs trisaccharide (A-tri, GalNAcα1,3[Fucα1,2]Gal) and blood group A type-2 tetrasaccharide (A-tetra, GalNAcα1,3[Fucα1,2]Galβ1,4GlcNAc) (a).1H NMR spectrum shows the anomeric protons of A-tri at 305 K (b). Structures of the different A-tri forms and their distribution in solution at 305 K (c). Figure 1: Structures and NMR spectra of A-tri and A-tetra glycans. Structures of A-type HBGAs trisaccharide (A-tri, GalNAcα1,3[Fucα1,2]Gal) and blood group A type-2 tetrasaccharide (A-tetra, GalNAcα1,3[Fucα1,2]Galβ1,4GlcNAc) ( a ). 1 H NMR spectrum shows the anomeric protons of A-tri at 305 K ( b ). Structures of the different A-tri forms and their distribution in solution at 305 K ( c ). Full size image We have used Saturation Transfer Difference (STD) NMR spectroscopy to study the interaction of rotavirus VP8* protein and A-type HBGAs. This NMR method is based on the transfer of saturation from the protein to bound ligands that are in fast exchange with a binding site, and therefore allows the discrimination of binding and non-binding ligands. The degree of saturation a ligand proton receives from the target protein can be directly translated into a ligand-binding epitope. Ligand protons that are in close contact to the protein surface receive larger saturation and will therefore produce larger STD NMR effects compared to protons that are more solvent exposed [28] , [29] . We obtained the 1 H NMR spectrum of A-tri ( Fig. 2a ) and the control STD NMR spectra of A-tri with glutathione- S -transferase (GST) ( Fig. 2b ) and A-tri in complex with recombinantly expressed GST-tagged VP8* from human rotavirus strains Wa, K8 and HAL1166. The STD NMR spectrum of GST-Wa VP8* in complex with A-tri showed no recognition of A-tri ( Fig. 2c ). However, the STD NMR spectra of GST-K8 VP8* ( Fig. 2d ) and GST-HAL1166 VP8* ( Fig. 2e ) in complex with A-tri unequivocally show that both proteins bind to A-tri. The control STD NMR spectrum of the GST fusion tag alone with A-tri shows no significant signal intensities, confirming that A-tri does not interact with GST. It is worth noting that this important control STD NMR spectrum demonstrates that all observed signals in the spectra of HAL1166 and K8 VP8* originate from binding of A-tri to VP8*. The strongest interaction of A-tri was observed for the methyl protons of the GalNAc N -acetamido group (NHAc, δ =1.73 p.p.m.) for both Hal1166 and K8 VP8* proteins. No STD NMR signal was observed for the H-disaccharide (Fucα1,2Galβ), emphasizing the significance of the GalNAc moiety for A-tri binding to HAL1166 ( Supplementary Fig. 1 ). It is most striking that STD NMR signals were also observed for the GalNAc H2 proton of two A-tri species: A-tri p α and A-tri p β . In addition, the H4 proton of the galactose moiety also received saturation for A-tri p α and A-tri p β . However, the X-ray crystal structure of A-tri with HAL1166 VP8* revealed that only the pyranose α-anomer, a biologically irrelevant configuration, binds to the protein [23] . In HBGA precursors, the glycosidic linkage between Gal and GlcNAc is always a β-configuration. Our solution binding study demonstrates that A-tri p α and A-tri p β are able to bind to K8 and HAL1166 VP8*, and that the binding epitope of A-tri for both proteins is identical, suggesting the same binding mode of A-tri, irrespective of the reducing end ( Supplementary Fig. 2a,b ). A homology model of K8 VP8* was generated using the HAL1166 VP8* X-ray crystal structure (pdb accession code: 4DRV [23] ) ( Supplementary Fig. 3 ) with a sequence identity of 83.9% and sequence similarity of 90.7%. The binding-site residues show minor variations supporting the identical binding epitope of A-tri determined by STD NMR experiments. 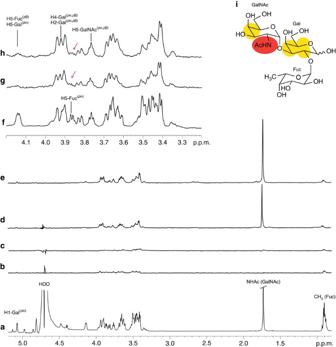Figure 2: NMR spectra of A-tri complexed with K8, HAL1166 and Wa VP8*. 1H NMR (a) and STD NMR (b–f) of human VP8* with A-type HBGA trisaccharide (A-tri, GalNAcα1,3[Fucα1,2]Gal) in 70 mM phosphate buffer pH 7.1 and 50 mM NaCl at 280 K. In detail, STD NMR spectra are shown for 24 μM GST and 2.4 mM A-tri (b), 18 μM GST-Wa VP8* and 1.8 mM A-tri (c), 36 μM GST-K8 VP8* and 2.4 mM A-tri (d), 24 μM GST-HAL1166 VP8* and 2.4 mM A-tri (e). Expansion of the spectrum from 4.2 to 3.2 p.p.m. is shown for the1H NMR (f) and STD NMR spectra of 36 μM GST-K8 VP8* and 2.4 mM A-tri (g) and 24 μM GST-HAL1166 VP8* and 2.4 mM A-tri (h). Epitope map of A-tri when bound to K8 and HAL1166 VP8*: red, strong STD NMR effects; yellow weak STD NMR effects (i). Figure 2: NMR spectra of A-tri complexed with K8, HAL1166 and Wa VP8*. 1 H NMR ( a ) and STD NMR ( b–f ) of human VP8* with A-type HBGA trisaccharide (A-tri, GalNAcα1,3[Fucα1,2]Gal) in 70 mM phosphate buffer pH 7.1 and 50 mM NaCl at 280 K. In detail, STD NMR spectra are shown for 24 μM GST and 2.4 mM A-tri ( b ), 18 μM GST-Wa VP8* and 1.8 mM A-tri ( c ), 36 μM GST-K8 VP8* and 2.4 mM A-tri ( d ), 24 μM GST-HAL1166 VP8* and 2.4 mM A-tri ( e ). Expansion of the spectrum from 4.2 to 3.2 p.p.m. is shown for the 1 H NMR ( f ) and STD NMR spectra of 36 μM GST-K8 VP8* and 2.4 mM A-tri ( g ) and 24 μM GST-HAL1166 VP8* and 2.4 mM A-tri ( h ). Epitope map of A-tri when bound to K8 and HAL1166 VP8*: red, strong STD NMR effects; yellow weak STD NMR effects ( i ). Full size image We have also analysed interactions of A-tri with VP8* proteins from P[6] (RV-3) and P[4] (DS-1) human rotaviruses. A-tri binding affinity to RV-3 and DS-1 was identified ( Fig. 3b,c , respectively), with a strong STD NMR signal observable for the N -acetamido group of the GalNAc residue. Strikingly, the methyl group of the fucose moiety (CH 3 Fuc, ~1 p.p.m.) shows the most predominant STD NMR signal intensity, leading to the conclusion that the fucose moiety of A-tri does interact with the VP8* protein of DS-1 and RV-3. Our NMR study provides the first detection of a direct interaction of the HBGA fucose moiety with any rotavirus VP8* protein. However, absolute STD NMR signal intensities were substantially lower compared with the spectra acquired for A-tri in complex with HAL1166 and K8. To validate protein activity, an equimolar concentration of GM1a glycan, a confirmed receptor for the DS-1-like P[4] rotavirus strain RV-5 and for RV-3 (ref. 22 ) was added to the A-tri complex of VP8* protein from DS-1 or RV-3. 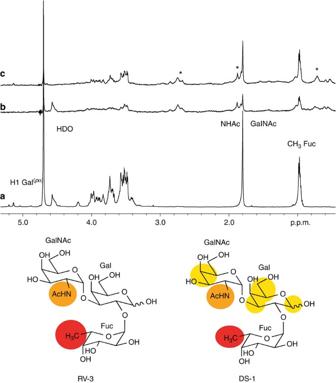Figure 3: NMR spectra of A-tri complexed with RV-3 and DS-1 VP8*. 1H NMR (a) and STD NMR (b,c) of human VP8* with A-type HBGA trisaccharide (A-tri, GalNAcα1,3[Fucα1,2]Gal) in 70 mM phosphate buffer pH 7.1 and 50 mM NaCl at 280 K. In detail, STD NMR spectra are shown for 24 μM GST-RV-3 and 2.4 mM A-tri (b), and 24 μM GST-DS-1 VP8* and 2.4 mM A-tri (c). Epitope map of A-tri when bound to RV-3 and DS-1 VP8* are shown in the lower panel VP8*: red, strong STD NMR effects; orange, medium STD NMR effects; yellow, weak STD NMR effects (*=protein background signals). Figure 3: NMR spectra of A-tri complexed with RV-3 and DS-1 VP8*. 1 H NMR ( a ) and STD NMR ( b , c ) of human VP8* with A-type HBGA trisaccharide (A-tri, GalNAcα1,3[Fucα1,2]Gal) in 70 mM phosphate buffer pH 7.1 and 50 mM NaCl at 280 K. In detail, STD NMR spectra are shown for 24 μM GST-RV-3 and 2.4 mM A-tri ( b ), and 24 μM GST-DS-1 VP8* and 2.4 mM A-tri ( c ). Epitope map of A-tri when bound to RV-3 and DS-1 VP8* are shown in the lower panel VP8*: red, strong STD NMR effects; orange, medium STD NMR effects; yellow, weak STD NMR effects (*=protein background signals). Full size image Quantitative analysis of the HAL1166 VP8*-A-tri STD NMR spectra revealed that the fucose residue of A-tri does not receive any saturation via the protein. This solution-based observation is in excellent agreement with the reported X-ray crystal structure [23] , where the fucose moiety does not make intimate contact with the protein. However, this finding raises the question of how important HBGAs are as receptors for P[III] rotavirus infection, as the fucose residue is the carbohydrate determinant that defines the ABH and Lewis antigens [30] . An interesting and relevant comparison is with another clinically significant human gastrointestinal virus, norovirus. All major genogroups of human norovirus have a clear dependence on HBGAs for infectivity and exhibit a relatively broad binding specificity for A, B, H or Lewis antigens [31] , [32] . Furthermore, a recent study has led to the proposal that HBGA-like substances associated with human enteric bacteria bind human norovirus and may have an impact on transmission and infection of this virus [33] . Interestingly, crystallography studies revealed that norovirus predominantly interacts with the fucose moiety of the blood group antigens [34] , [35] , [36] , [37] . In fact, the α1,3- and α1,4-fucose residues of Lewis HBGAs are claimed to be essential for binding to GII.4 noroviruses [36] , [37] . STD NMR studies on GII.4 virus-like particles derived from norovirus Ast6139 underlined the broad HBGA-binding profile of GII.4 noroviruses. A, B, H and Lewis epitopes, with and without a sialic acid, are recognized by norovirus-like particles, leading to the conclusion that the minimal recognition unit for norovirus was α- L -fucose [38] . Our study herein shows that the fucose moiety is irrelevant for blood group antigen binding to the investigated P[III] rotavirus spike proteins. Clearly, if P[III] rotavirus infection depended on the A, B, H and Lewis blood groups, an engagement of the key sugar residue, fucose, with the viral protein would be anticipated. Although our study indicates that fucose plays no direct role in the recognition event, it does not rule out that it may still play an indirect role in stabilizing the blood group antigen through non-conventional hydrogen bonds as has recently been described for Lewis x (ref. 39 ). Our study also demonstrates a lack of A-tri recognition by VP8* from the clinically relevant human P[8, II] rotavirus Wa. We identified that GM1a glycan bound as expected to the A-tri complex of Wa VP8* and the Wa VP8* competed with Wa virus for infectivity, confirming protein function. Moreover, using STD NMR spectroscopy no recognition of H type-1 and Lewis b antigens by the P[8] Wa VP8* was observed ( Supplementary Fig. 4 ). In contrast, a recent study based on assays for VP8* binding to human saliva and synthetic oligosaccharides led to the conclusion that H type-1 and Lewis b antigens can interact with Wa VP8* (ref. 25 ). Notably, the Wa strain represents an important current and past lineage of the most common human rotavirus serotype worldwide [40] but shows only 43% VP8* sequence identity with HAL1166, and most of the amino acids in the glycan-binding site differ substantially ( Supplementary Fig. 5 ). Importantly, our present study demonstrates for the first time that VP8* of DS-1 and RV-3 rotaviruses recognize A-tri. After P[8,II], these viruses represent the next most common genotypes P[4,II] and P[6,II], and show relatively low VP8* sequence identity to HAL1166 (44 and 47%, respectively). Significantly, the A-tri engagement with VP8* from both DS-1 and RV-3 involves the fucose moiety. This fucose recognition is consistent with a recent study in children from Burkina Faso, which showed an association of P[6] rotavirus disease predominantly with a Lewis-negative phenotype, independent of secretor status [41] . A-tetra and A-tri have an identical binding epitope for K8 and HAL1166 VP8* We have also used STD NMR spectroscopy to investigate the VP8* interaction of the biologically relevant A type-2 HBGAs tetrasaccharide (A-tetra), which has an additional GlcNAc residue ( Fig. 4a–g ). The initial 1 H NMR spectrum of A-tetra shows no distinct forms as in the case of A-tri ( Fig. 4a ). A control STD NMR experiment of the GST fusion tag in the presence of A-tetra shows no significant STD NMR signals ( Fig. 4b ), confirming that all STD NMR signals for A-tetra in complex with GST-K8 VP8* ( Fig. 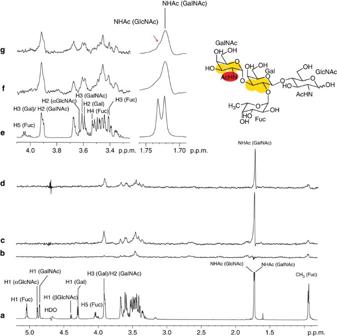Figure 4: NMR spectra of A-tetra complexed with K8 and HAL1166 VP8*. 1H NMR (a) and STD NMR (b–d) of human VP8* with A HBGA type-2 tetrasaccharide (A-tetra, GalNAcα1,3[Fucα1,2]Galβ1,4GlcNAc) in 70 mM phosphate buffer pH 7.1 and 50 mM NaCl at 280 K. In detail, STD NMR spectra are shown for 24 μM GST and 2.4 mM A-tetra (b), 24 μM GST-K8 VP8* and 2.4 mM A-tetra (c), 24 μM GST-HAL1166 VP8* and 2.4 mM A-tetra (d). Expansion of the spectrum from 4.1 to 3.3 p.p.m. is shown for the1H NMR (e) and STD NMR of 24 μM GST-K8 VP8* and 2.4 mM A-tetra (f), and 24 μM GST-HAL1166 VP8* and 2.4 mM A-tetra (g). Epitope map of A-tetra when bound to K8 and HAL1166 VP8*: red, strong STD NMR effects; yellow, weak STD NMR effects (h). 4c,f ) and GST-HAL1166 VP8* ( Fig 4d,g ) are genuine and are derived from the binding of A-tetra to VP8* and not GST. Similar to A-tri recognition, the N -acetamido group’s methyl protons of the crucial A-tetra GalNAc moiety (NHAc, δ =1.72 p.p.m.) received the highest saturation, implying a very close contact with the protein surface. However, our STD NMR studies demonstrated that the additional GlcNAc residue N -acetamido group methyl protons do not engage with either HAL1166 VP8* ( Fig. 4g ) or K8 ( Fig. 4f ). Furthermore, the GalNAc, and Gal H2 and H3 protons also show strong STD NMR signals, whereas the ring protons of the GlcNAc residue do not produce significant STD NMR signals. The fucose residue is entirely solvent exposed and does not interact with the protein. Therefore, we conclude that the binding epitope of A-tetra is identical to that of A-tri when complexed with HAL1166 VP8*. Finally, from this study we have discovered that the binding epitopes of A-tri and A-tetra are also identical when bound to K8 VP8*, with only very small differences observed in STD NMR signal intensities ( Supplementary Fig. 2 ). Figure 4: NMR spectra of A-tetra complexed with K8 and HAL1166 VP8*. 1 H NMR ( a ) and STD NMR ( b–d ) of human VP8* with A HBGA type-2 tetrasaccharide (A-tetra, GalNAcα1,3[Fucα1,2]Galβ1,4GlcNAc) in 70 mM phosphate buffer pH 7.1 and 50 mM NaCl at 280 K. In detail, STD NMR spectra are shown for 24 μM GST and 2.4 mM A-tetra ( b ), 24 μM GST-K8 VP8* and 2.4 mM A-tetra ( c ), 24 μM GST-HAL1166 VP8* and 2.4 mM A-tetra ( d ). Expansion of the spectrum from 4.1 to 3.3 p.p.m. is shown for the 1 H NMR ( e ) and STD NMR of 24 μM GST-K8 VP8* and 2.4 mM A-tetra ( f ), and 24 μM GST-HAL1166 VP8* and 2.4 mM A-tetra ( g ). Epitope map of A-tetra when bound to K8 and HAL1166 VP8*: red, strong STD NMR effects; yellow, weak STD NMR effects ( h ). Full size image A-tri adopts a different conformation when bound to K8 VP8* The conformation of glycans when bound to proteins (bioactive conformation) can significantly vary in solution compared with a single conformation obtained with X-ray crystallography. To determine the bioactive conformation of A-tri when bound to VP8* in solution, we acquired Nuclear Overhauser Enhancement spectroscopy (NOE) NMR spectra of free A-tri in solution and transferred NOE (trNOE) NMR experiments of A-tri in complex with K8 VP8* following a similar approach to that previously reported [11] . The NOE NMR spectrum shows that A-tri has positive NOEs (diagonal and cross-signals of opposite sign) at a temperature of 305 K ( Fig. 5a ). On the contrary, the trNOE experiment of a VP8* K8:A-tri-complex ( Fig. 5b ) at a 1:10 (protein:ligand) molar ratio clearly indicate that the NOEs are negative, leading to the assumption that A-tri has adopted the rotational correlation time ( τ c ) of the VP8* due to association with the protein. Conversely, the trNOE experiment of A-tri in complex with Wa VP8* does not result in a change of the sign of NOE signals, indicating that A-tri has no binding affinity for Wa VP8* ( Fig. 5c ). The observed reduced intensity of the NOE signal ( Fig. 5c ) can be explained by a substantially lower ligand concentration in the trNOE compared with the NOE experiment of the free ligand in solution. A more detailed comparison between the NOE and trNOE spectra indicates significant differences in the NOE pattern. Most striking is the disappearance of the interglycosidic NOE between the fucose methyl group, the CH 3 (Fuc) residue and the H1 (Gal) proton of bound A-tri. This particular NOE shows a strong signal in the uncomplexed NOE spectrum ( Fig. 5a ), indicating that the bioactive conformation of A-tri must be different to the predominant solution conformation adopted in the absence of the protein. The disappearance of a crucial NOE can be explained by a conformational rearrangement of the ligand on binding to the protein, most probably around the α1,2-glycosidic linkage between the fucose and galactose residue. This is in excellent agreement with the binding epitope obtained from STD NMR experiments, revealing that the fucose is not engaged with the protein and remains solvent exposed, resulting in a higher degree of flexibility. 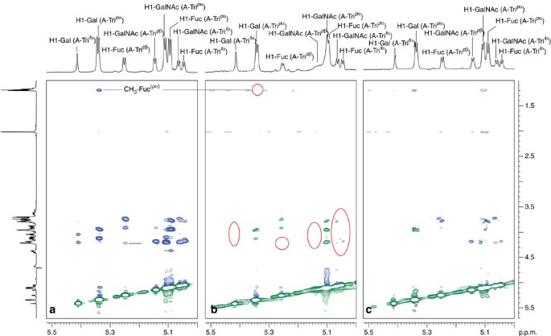Figure 5: NOE of A-tri and trNOE spectra of A-tri in complex with K8 VP8*. NOE of A-type HBGA trisaccharide (A-tri, GalNAcα1,3[Fucα1,2]Gal) in aqueous solution at a mixing timeτmof 800 ms (a). Transferred NOE (trNOE) of A-tri in a complex with rotavirus K8 VP8* (b) and Wa VP8* (c), respectively, at a ratio of 1:12 (protein:ligand) and a mixing timeτmof 150 ms. NOE spectrum (b) indicates binding due to strong negative NOE’s, whereas spectrum (c) indicates no binding due to the occurrence of small positive NOEs. Figure 5: NOE of A-tri and trNOE spectra of A-tri in complex with K8 VP8*. NOE of A-type HBGA trisaccharide (A-tri, GalNAcα1,3[Fucα1,2]Gal) in aqueous solution at a mixing time τ m of 800 ms ( a ). Transferred NOE (trNOE) of A-tri in a complex with rotavirus K8 VP8* ( b ) and Wa VP8* ( c ), respectively, at a ratio of 1:12 (protein:ligand) and a mixing time τ m of 150 ms. NOE spectrum ( b ) indicates binding due to strong negative NOE’s, whereas spectrum ( c ) indicates no binding due to the occurrence of small positive NOEs. Full size image Molecular dynamics simulation reveals flexibility of the fucose residue To further confirm the flexibility of the fucose residue, molecular dynamics (MD) simulation of A-tri p α in complex with HAL1166 ( Supplementary Fig. 6 ) was conducted based on the X-ray crystal structure (pdb 4DRV) [23] . Our MD simulation reveals that the α1,2-glycosidic linkage between the fucose and galactose residue is highly flexible. Furthermore, our simulation indicates that this linkage can easily adopt a conformation where the intermolecular distance between the H1 (Gal) and CH 3 (Fuc) is >4.0 Å. A-tri conformations (63.4%) before reaching energy equilibrium (~1 ns) show a shorter distance between H1 (Gal) and CH 3 (Fuc) (1.8–4.0 Å). However, after reaching equilibrium the MD simulation revealed that only 9.4% of all A-tri conformations indicate a shorter distance (1.8–4.0 Å) and the majority (90.6%) of all conformations reveal a larger distance between the H1 Gal and CH 3 Fuc (>4.0 Å) that would not result in the detection of an NOE. This distance calculation is in excellent agreement with the trNOE experimental outcomes that show a complete disappearance of this important NOE. The VP8* engagement of A-tri p α is mainly through the GalNAc moiety and the non-binding fucose residue appears to have a high degree of rotational freedom. Another important observation is that negative NOEs, clear evidence of binding, could not be detected for A-tri with the galactose adopting a furanose form (A-tri f α ); hence, it has no binding affinity. This result is not surprising as hexofuranosyl residues are absent in mammalian glycoconjugates and only found in oligo- and polysaccharides of bacteria, protozoa, fungi, plants and archaebacteria [42] . This finding is further supported by STD NMR experimental analysis that shows VP8* can only accommodate A-tri when the internal galactose residue adopts a biologically relevant pyranose form. Interestingly, the observed severe line broadening for the H1 (GalNAc) signals for both pyranose α - and β -anomers (A-tri p α and A-tri p β ) suggests close protein interaction and is in excellent agreement with the determined A-tri glycointeractome by STD NMR spectroscopy (see Fig. 2 ). Specificity and affinity of A-type HBGA binding to VP8* To quantify the affinity of A-tri and A-tetra when bound to rotavirus VP8* protein, we have determined K D -values using 1 H– 15 N heteronuclear single quantum correlation (HSQC) chemical shift perturbation NMR experiments [43] , [44] . Upon addition of the ligand to uniformly 15 N-labelled VP8* protein, changes in 1 H and 15 N chemical shifts can only be detected for those backbone amides that are in close contact with the ligand. A K D -value of 1.2 mM has been previously reported using the same approach for the sialidase-sensitive rhesus rotavirus (RRV) VP8* protein and 3′-sialyllactose as ligand [14] . In the current study, we have determined the K D -values for A-tri and A-tetra following the glycan induced chemical shift perturbations of the backbone amides of K8 and HAL1166 VP8* for ten residues that show the strongest changes ( Fig. 6 ). A complete 1 H– 15 N HSQC spectral analysis of these perturbations was undertaken ( Supplementary Figs 7–9 ). We found that the affinity of A-tri is significantly stronger for HAL1166 VP8* ( K D 1.5 mM) compared to K8 VP8* ( K D 3.4 mM). Interestingly, the blood group-A tetrasaccharide (A-tetra) showed lower K D values when bound to HAL1166 and K8 VP8*, of 0.8 and 1.7 mM, respectively ( Fig. 6 ). This can be explained by the fact that A-tetra does not adopt α,β-anomeric mixtures of both the pyranose and furanose forms in solution as does A-tri where only the α- and β-pyranose forms of Gal showed binding affinity to VP8* and not the α- and β-furanose forms. Nevertheless, A-tetra also shows a higher affinity for HAL1166 VP8* over K8 VP8*. No changes in the total number of chemical shift perturbations were identified for protein complexes with A-tetra compared to A-tri. This confirms the STD NMR outcomes that the additional GlcNAc residue does not interact with the protein and that the binding epitopes of A-tri and A-tetra are identical ( Supplementary Figs 8 & 9 ). No significant chemical shift perturbations were observed for human rotavirus Wa VP8* in the presence of A-tri (58 mM), providing further evidence that A type HBGAs do not bind to Wa VP8* ( Supplementary Fig. 10 ). Interestingly, addition of Lewis b even at a very high concentration (19.7 mM), to 15 N-labelled Wa VP8* also did not result in any chemical shift perturbations. These results are in agreement with our STD NMR results and indicate that Lewis b does not bind to VP8*. 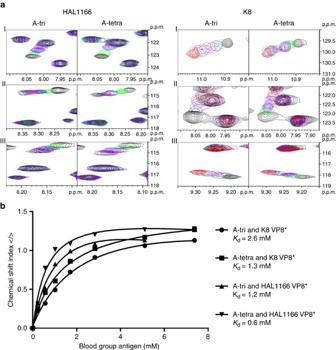Figure 6:15N HSQC NMR spectra of A-tri in complex with HAL1166 and K8 VP8*. 1H–15N HSQC NMR titration of A-type HBGA trisaccharide (A-tri) and A- type-2 HBGA tetrasaccharide (A-tetra) binding to 0.4 mM HAL1166 and 0.4 mM K8 VP8*. Overlayed spectra of all titration steps are shown for the three strongest amide shifts (I, II, III;a). Dissociation constants (Kd) were obtained by nonlinear regression based on a single binding site model fitting the chemical shift index <I> as an average of the ten strongest amide shifts (b). Figure 6: 15 N HSQC NMR spectra of A-tri in complex with HAL1166 and K8 VP8*. 1 H– 15 N HSQC NMR titration of A-type HBGA trisaccharide (A-tri) and A- type-2 HBGA tetrasaccharide (A-tetra) binding to 0.4 mM HAL1166 and 0.4 mM K8 VP8*. Overlayed spectra of all titration steps are shown for the three strongest amide shifts (I, II, III; a ). Dissociation constants ( K d ) were obtained by nonlinear regression based on a single binding site model fitting the chemical shift index < I > as an average of the ten strongest amide shifts ( b ). Full size image A-Tri blocks cell binding by VP8* of HAL1166 but not Wa To corroborate our NMR and molecular modeling results, we have investigated if A-tri blocks VP8* binding to highly rotavirus-permissive MA104 cells ( Fig. 7a , Supplementary Fig. 11 ). Using flow cytometry, we have demonstrated significant levels of cell binding by VP8* of HAL1166 ( P =0.0005), K8 ( P =0.0060) and Wa ( t -test, P <0.0001) over the background (control) binding. Treatment with 2 mM and 10 mM A-tri reduced the specific cell binding of HAL1166 VP8* by 53% ( t -test, P =0.0074) and 69% ( t -test, P =0.021), respectively, but had no effect on specific cell binding by K8 VP8* ( t -test, P >0.22) or Wa VP8* ( t -test, P >0.05). The increased level of HAL1166 VP8* cell binding compared with K8 VP8*, and the dose-dependent A-tri blockade of HAL1166 but not K8 VP8* binding, can be explained by the higher K D -value of A-tri for K8 VP8* than HAL1166 VP8* ( Fig. 6 ). 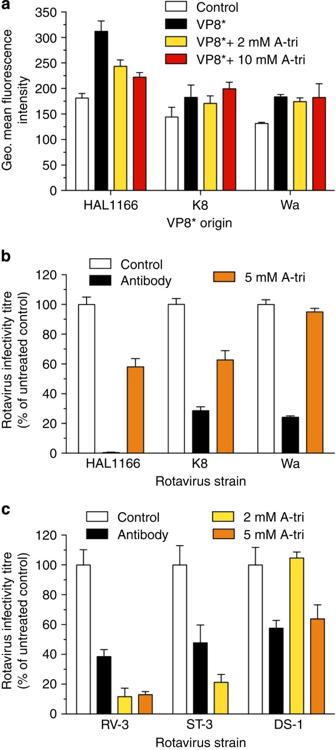Figure 7: A-tri competition with cell binding by rotavirus VP8* and rotavirus infection. Effect of A-type HBGA trisaccharide (A-tri, GalNAcα1,3[Fucα1,2]Gal) on MA104 cell binding by VP8* of rotaviruses HAL1166, K8 and Wa (a), the infectivity of these rotaviruses (b) and the infectivity of P[6] rotaviruses RV-3 and ST-3, and P[4] rotavirus DS-1 (c). The effect of rotavirus treatment with 2 mM or 5 mM A-tri on infectivity was determined. Neutralizing antibodies (Antibody) used as positive controls were B37:1 (HAL1166), RV-4:3 (K8), 1A10 (Wa), RV-3:1 (RV-3), ST-3:3 (ST-3) and RV-5:2 (DS-1). Three replicates were analysed for each condition. The data shown are representative of the findings of two independent experiments. Bars indicate the s.d. Figure 7: A-tri competition with cell binding by rotavirus VP8* and rotavirus infection. Effect of A-type HBGA trisaccharide (A-tri, GalNAcα1,3[Fucα1,2]Gal) on MA104 cell binding by VP8* of rotaviruses HAL1166, K8 and Wa ( a ), the infectivity of these rotaviruses ( b ) and the infectivity of P[6] rotaviruses RV-3 and ST-3, and P[4] rotavirus DS-1 ( c ). The effect of rotavirus treatment with 2 mM or 5 mM A-tri on infectivity was determined. Neutralizing antibodies (Antibody) used as positive controls were B37:1 (HAL1166), RV-4:3 (K8), 1A10 (Wa), RV-3:1 (RV-3), ST-3:3 (ST-3) and RV-5:2 (DS-1). Three replicates were analysed for each condition. The data shown are representative of the findings of two independent experiments. Bars indicate the s.d. Full size image A-tri inhibits infection by K8, HAL1166, RV-3, ST-3 and DS-1 but not Wa The effect of A-tri treatment on MA104 cell infection by a range of human rotaviruses was determined. All of these viruses were passaged to a similar low extent. Infectivity measurements were more sensitive than VP8*-cell binding assays for the detection of A-tri use, as a 37% decrease in K8 infectivity following exposure to 5 mM A-tri was observed ( P =0.0009; Fig. 7b ). As expected from the increased HAL1166 infectivity in cells genetically modified to express A-tri (ref. 23 ), the infectivity of HAL1166 in MA104 cells was inhibited by 42% after A-tri exposure ( t -test, P <0.0001). In contrast, the presence of A-tri did not alter Wa infectivity ( t -test, P =0.09; Fig. 7b ), in excellent agreement with our NMR results. Overall, we have observed that K8 rotavirus is less dependent on A-type antigen for VP8*-cell binding than HAL1166, and shows a similar dependence on this antigen to HAL1166 for infectivity. In contrast, Wa rotavirus does not recognize this antigen. Consistent with the A-tri recognition of the VP8* of DS-1 and RV-3 detected by STD NMR ( Fig. 3 ), A-tri at 5 mM inhibited the infectivity of DS-1 and RV-3 rotaviruses, by 36% ( t -test, P =0.001) and 87% ( t -test, P <0.0001), respectively ( Fig. 7c ). Infectivity blockade was still evident at 2 mM A-tri for RV-3 (88%; t -test, P <0.0001) and another P[6] human rotavirus ST-3 (79%; t -test, P <0.0001), but not DS-1 ( Fig. 7c ). H type-1 and Lewis b HBGA do not inhibit P[II]/[III] viruses We could not detect any blockade of HAL1166, K8 or Wa rotavirus infectivity by H type-1 and Lewis b antigen at a 10 mM concentration ( Supplementary Fig. 12 ). This is supported by both STD NMR and 1 H– 15 N HSQC chemical shift perturbation NMR experiments, which revealed no H type-1 and Lewis b antigen recognition by HAL1166, K8 or Wa rotavirus VP8* ( Supplementary Figs 1, 4 and 10 ). Similarly, 10 mM H type-1 or Lewis b antigen did not affect the infectivity of RV-3, ST-3 or DS-1 ( Supplementary Fig. 12 ). From the presented data determined by our multidisciplinary receptor studies, using recombinant VP8* and whole viruses, we conclude that HBGAs play a role in human rotavirus infection of host cells but substantial virus strain-specific variations in HBGA usage are evident. The A-type HBGAs show some interaction with the P[III] HAL1166 strain but may be less important for P[III] K8 rotavirus. For these rotaviruses, the histo-blood group-specific fucose moiety did not interact with VP8*. Furthermore, other related fucosylated glycans such as Lewis b and H type-1 antigen neither bind to HAL1166 and K8 VP8* nor facilitate infection by these viruses. We have also demonstrated that A-type HBGAs, Lewis b antigen and H type-1 antigen neither bind to Wa VP8* nor facilitate infection by Wa, which is a representative of an important current and past lineage within the most common disease-causing P[II] human rotaviruses [40] . It is a reasonable assumption that a rotavirus strain such as Wa, representing a major P[8] rotavirus lineage, might become prevalent partly because it does not discriminate between hosts according to their secretor status. We also found that Lewis b and H type-1 antigens do not inhibit infection by other P[II] human rotaviruses, including DS-1 (P[4]) and ST-3 (P[6]), whose VP8* were previously reported to bind one or both of these antigens [25] . We have discovered that A-type HBGA interacts with the VP8* of human P[4] and P[6] rotaviruses. In these complexes, we determined, for the first time, an involvement of the fucose moiety with the protein surface. This engagement may help explain why A-tri reduces infection by P[6] rotavirus RV-3 more substantially than the P[14] HAL1166 and P[9] K8 strains. However, as the DS-1 infectivity reduction by A-tri was similar to that of HAL1166 and K8, other factors are also likely to be involved, including the difference in usage of other receptors such as integrins between DS-1 and RV-3 (ref. 45 ). Taken together, our data revealed that HBGAs are used as rotavirus receptors, consistent with their abundance on the surface of mucosal epithelia of the gastrointestinal tract. However, it is notable that major rotavirus strain variations in HBGA recognition were detected. The relevant human clinical strain Wa did not recognize HBGAs, which is consistent with the observed lack of influence of genetically controlled expression of different HBGAs on pediatric rotavirus gastroenteritis [46] , [47] . Interestingly, two recent studies suggested that non-secretor individuals (null homozygote fucosyltransferase, FUT2) are not susceptible to infection with the most common rotaviruses [48] , [49] . However, this finding appears inconsistent with the well-established fact that by 2–3 years of age, essentially all children excrete rotavirus at least once and/or seroconvert to rotavirus regardless of their secretor status [50] , [51] . Although only a small number of children were analysed, a further recent study [41] may shed light on this discrepancy with its finding that non-secretors may be preferentially infected by P[6] rather than P[8] rotaviruses. This also indicates that all children are susceptible to rotavirus infection, independent of their blood group. Consequently, the interdependence of rotavirus infection and disease on secretor status remains questionable. The possibility that rotaviruses, such as noroviruses, may bind HBGA-like substances on intestinal bacteria also should be considered [33] , [52] , especially in the light of recent evidence that antibiotic treatment reduces rotavirus infection [53] . The complex regulation of fucosylation by FUT2 on intestinal epithelium, proposed to be controlled by innate lymphoid cells and involve IL-22 induction by commensal bacteria [54] , [55] also may contribute to the apparent inconsistencies between studies of the roles of HBGA in rotavirus receptor usage and disease. Our study indicates that HBGA play a role in host cell invasion by several human rotavirus genotypes. However, the clear differences we found between rotavirus strains in their ability to use HBGA show that HBGA may not be essential in this process. In this context, it is important to note that FUT2 activity is not restricted to the biosynthesis of H type-1 precursors (Galβ1,3GlcNAc). Glycolipids in the epithelial tissues of the gastrointestinal tract are also fucosylated [56] by FUT2. Clearly, secretor status of the individual and FUT2 enzyme activity are not correlated with blood group specificity. More extensive structural, virological and epidemiological studies are required to shed light on the exact role played by HBGAs in rotavirus infection and disease. Viruses and cells The origins of human rotaviruses HAL1166, K8, Wa, RV-3, ST-3 and DS-1 have been described previously [45] , [57] , [58] . These viruses were cultivated in the MA104 monkey kidney cell line (ATCC CRL-2378) using DMEM containing 2 mM L-glutamine (Sigma-Aldrich), 20 mM HEPES (Roche) and antibiotics (DMEM) supplemented with 10% (v/v) fetal bovine serum. Rotavirus infectivity was activated with porcine pancreatic trypsin (Sigma) at 20 μg ml −1 for 20 min at 37 °C, and infectivity assays were performed as before [45] , [57] . Carbohydrates and reagents Deuterium oxide was purchased from Sigma Aldrich (Australia) and all glycans, that is A antigen trisaccharide (A-tri), A antigen tetrasaccharide (A-tetra), Lewis b and H type-1 antigens, were purchased from Elicityl (France). VP8* protein production Plasmids expressing the gene encoding the VP8* core proteins of HAL1166 (VP8* 64-224 ), K8 (VP8* 64-224 ), Wa (VP8* 64-223 ), RV-3 (VP8* 64-223 ) and DS-1 (VP8* 64-223 ) for NMR and rotavirus-binding assays were synthesized (HAL1166) or cloned from virus (Wa, K8, RV-3 and DS-1) as described previously for Wa (ref. 12 ). In brief, complementary DNA produced from viral dsRNA by reverse transcription was used as template for PCR with specific oligonucleotide primers ( Supplementary Table 1 ) to produce the VP8* gene fragment, which was cloned into the pGEX-4T-1 vector (GE Healthcare). DNA sequencing indicated that the predicted amino acid sequence of pGEX-Wa-VP8* was identical to the published Wa VP4 sequence [59] (GenBank accession code L34161 ), except for leucine substituting a phenylalanine as position 163; pGEX-K8-VP8* amino acid sequence was identical to the published sequence (GenBank accession code Q01641 ), except for a change from tyrosine to aspartic acid at amino acid position 149; and the sequence of pGEX-RV-3-VP8* [22] was identical to the most recent database entry for RV-3 VP4 (GenBank accession code FJ998273 ). Our sequence and FJ998273 both differ from the original published sequence (GenBank accession code U16299 ) in showing serine rather than proline at aa position 71 (refs 60 , 61 ). The pGEX-DS-1-VP8* amino acid sequence was identical to that published (GenBank accession code HQ650119 ). The VP8* gene fragment of HAL1166 was synthesized (GenScript) with 5′-BamH1 and 3′-EcoR1 restriction sites and ligated into the pUC57-Kan cloning vector through a single blunt-end EcoRV restriction site. Following digestion with BamH1 and EcoR1 of the pUC57-HAL1166-VP8* plasmid, the VP8* gene fragment was ligated into pGEX-4t-1, yielding pGEX-4t-1-HAL1166-VP8*. The final expression plasmid encoded for amino acids 64 to 224 of the VP4 protein and was fused to an N-terminal GST protein. For STD NMR, trNOE and cell-binding assays, the GST portion was not cleaved from the VP8* proteins. Protein expression was performed as described previously [19] . To prevent the formation of insoluble products, inclusion bodies and aggregates, the expression protocol was optimized for RV-3 VP8* by adding 20 ml l −1 of a 50 × stock solution of Augmedium (Athena Environmental Sciences, Inc., Baltimore, MD, USA), to precondition the cells and induce expression of chaperone proteins, followed by 30 min incubation. Isopropylthiogalactoside was added to reach a final concentration of 1 mM, to induce protein overexpression. Frozen cell pellets were thawed in PBS (137 mM NaCl, 2.7 mM KCl, 10 mM Na 2 HPO 4 , 2 mM KH 2 PO 4 pH 7.3) supplemented with 1 mM phenylmethylsulfonyl fluoride (Roche Diagnostics). The cells were lysed with 1 mg ml −1 lysozyme supplemented with 1% (w/v) Triton X-100 and 20 μg ml −1 DNaseI. Cell debris was removed by centrifugation at 20,000 g for 30 min and the supernatant was passed over a glutathione-Sepharose column (Amersham-Pharmacia Biotech). The column was washed with PBS-binding buffer and bound GST fusion protein was eluted with 50 mM Tris-HCl pH 7.4 supplemented with 10 mM glutathione. Expression of uniformly 15 N-labelled VP8* protein For the acquisition of 15 N– 1 H HSQC NMR experiments, HAL1166, K8 and Wa VP8* core proteins were expressed using 15 N-minimal growth medium. Cells were grown to OD 600nm =0.6 at 37 °C in common LB medium. Cells were pelleted and washed with 1 × M9 salts (22 mM KH 2 PO 4 , 45 mM Na 2 HPO 4 × H 2 O, 8.6 mM NaCl, pH 7.2) and then resuspended four times concentrated in 15 N-minimal growth medium (22 mM KH 2 PO 4 , 45 mM Na 2 HPO 4 × 7H 2 O, 8.6 mM NaCl, 18 mM 15 NH 4 Cl, 22 mM glucose, 2 mM MgSO 4 , 0.1 mM CaCl 2 , 1 × BME Vitamins pH 7.2) and incubated for 1 H at 25 °C before expression was induced by the addition of 0.1 mM isopropylthiogalactoside. Cells were harvested after 4 h. Purification including removal of the GST fusion protein was accomplished as previously described [19] . Standard NMR experiments Chemical shift assignment of A-Tri and A-Tetra in 20 mM deuterated phosphate buffer and 70 mM NaCl, pH 7.1, was achieved by COSY, TOCSY, HSQC, 1D NOESY and 1 H NMR experiments at 280 and 305 K. Chemical shift assignments were in agreement with published values [27] . STD NMR experiments All STD NMR spectra were acquired in Shigemi Tubes (Shigemi, USA) with a Bruker 600 MHz Avance spectrometer at 280 K using a conventional 1 H/ 13 C/ 15 N gradient cryoprobe system. NMR experiments of A-tri in complex with VP8*-GST protein and GST as a control experiment were prepared using a protein concentration of 24 or 36 μM and a ligand concentration of 2.4 mM, resulting in a total protein–ligand ratio of 1:100 and 1:67, respectively. The final volume was 200 μl containing 20 mM deuterated phosphate buffer and 70 mM NaCl, pH 7.1. The protein was saturated with a cascade of 40 Gaussian-shaped pulses with duration of 50 ms each at −0.1 p.p.m., resulting in a total saturation time of 2 s. The off-resonance was set to 33 p.p.m. and 1,024 experiments were acquired. A WATERGATE sequence was used to suppress the residual HDO signal. A spinlock filter with a strength of 5 kHz and duration of 10 ms was applied to suppress the protein background. NOE and trNOE NMR experiments NOE NMR experiments of free A-tri were acquired by diluting 1 mg of A-tri in 50 μl of 20 mM deuterated phosphate buffer and 70 mM NaCl, pH 7.1, at 305 K on a Bruker 600 MHz Avance spectrometer. The mixing time ( τ m ) was set to 800 ms and the relaxation delay to 2 s. trNOE NMR experiments were carried out using 1 mg GST-Wa or GST-K8, with a total molecular weight of 44 kDa and 145 μg of A-Tri that equals a protein:ligand ratio of 1:12 in 20 mM deuterated phosphate and 70 mM NaCl, pH 7.1, at 305 K and 600 MHz. The mixing time ( τ m ) for VP8*-GST protein was set to 150 ms to avoid false-positive NOEs due to spin diffusion effects. A trNOE NMR experiment of GST-K8 protein using the identical experimental setup but without ligand was acquired to subtract it from the trNOE with ligand to remove water background. 1 H- 15 N-HSQC NMR experiments To calculate solution dissociation constants ( K D ) of ligand, we used 1 H- 15 N-HSQC titration experiments, as was previously employed [15] . Using a standard 1 H- 15 N-HSQC NMR protocol, NMR spectra of 0.8 mM 15 N-labelled K8, HAL1166 and Wa VP8* were first acquired in the absence of ligand at 300 K on a 600-MHz NMR spectrometer equipped with a cryoprobe. The NMR buffer consisted of 20 mM Na 2 HPO 4 /NaH 2 PO 4 and 70 mM NaCl in 10% D 2 O. A-tri or A-tetra was titrated to the 15 N-labelled proteins in seven steps with 7.4 mM as the highest ligand concentration. 1 H- 15 N-HSQC spectra were acquired after each titration step, to follow the ligand-induced changes in the chemical shift perturbations of the protein backbone amide nitrogen and hydrogen. In a first analysis step, the amide shifts were calculated for the highest ligand concentration weighing proton shifts over nitrogen by a factor of five δ ( 1 H, 15 N)= δ ( 1 H)+ δ ( 15 N)/5 ( Supplementary Fig. 7 ). A threshold value of Δ δ ( 1 H, 15 N)=0.04 p.p.m. is considered as binding of the corresponding amino acid. Alternatively, this threshold is set to the s.d. of all chemical shifts. However, the full analysis shows that both alternative threshold values are very similar for the binding of A-tri and A-tetra to the VP8* proteins of the RV strains K8 and HAL1166 (s.d. for HAL1166 A-tri =0.036, HAL1166 A-tetra =0.042, K8 A-tri =0.037, K8 A-tetra =0.040; Supplementary Figs 8 and 9 ). Notably, the s.d. for the binding of A-tetra is slightly higher compared with A-tri. Binding affinities were calculated on the basis of the ten strongest backbone amide chemical shifts, which all showed a characteristic pattern of shift movements confirming the specificity of those changes ( Supplementary Figs 8 and 9 ). The chemical shifts were quantified by the chemical shift index for those strongly affected backbone amides according to the following formula: < I>= Σ{[( N 0 − N )/0.5] 2 +[( H 0 − H )/0.1] 2 } 1/2 , where N 0 and N are the amide 15 N chemical shifts in the absence and presence of ligand, respectively; H 0 and H are the backbone amide hydrogen chemical shifts in the absence and presence of ligand, respectively [11] . Calculations were performed using GraphPad Prism 6.0, by using nonlinear regression following a one-site total binding model according to < I >= B max *[A-tri]/( K d +[A-tri])+NS*[A-tri]+Background, with B max the maximum specificity binding and NS the slope of nonspecific binding. Homology modelling of K8 VP8* A homology model of K8 VP8* protein was built using the X-ray crystal structure HAL1166 X (pdb accession code: 4DS0 ) as template using YASARA Structure molecular modelling package (Ver. 13.9.8) [62] ( Supplementary Fig. 5 ). The HAL1166 structure (pdb code: 4DRV [23] ) was chosen as a suitable template, as it has a sequence identity of 83.9% and sequence similarity (BLOSUM62 score is >0) of 90.7%. The subsequent, fully unrestrained simulated annealing minimization, run for the entire model, resulted in an overall quality Z -score of −0.081 and indicates a high-quality homology model. Both proteins share the amino acid sequence (Ser187-Tyr188-Leu189-Leu190-Thr191) that has been identified as containing key residues for HBGA binding in the case of HAL1166 VP8* [23] . After the side chains had been built, optimized and fine-tuned, all newly modelled parts were subjected to a combined steepest descent and simulated annealing minimization (that is, the backbone atoms of aligned residues were kept fixed to avoid potential damage. The hm_build.mcr macro of the YASARA package with default parameters was used. MD simulations To analyse the flexibility of the α(1,2)-glycosidic linkage of A-tri, the three-dimensional structure HAL1166 VP8* protein in complex (pdb 4DRV) [23] a 2.8Ns MD calculation was performed using the YASARA Structure molecular modeling package (Ver. 13.9.8). The model was subjected to further refinement using the md_refine.mcr macro using the AMBER99 force field. Simulation parameters were kept at the values defined by the macro. Flow cytometric analysis of VP8*-cell binding Binding by GST-VP8* from HAL1166, K8 and Wa rotaviruses to MA104 cells was assayed in the same experiment at 4 °C as previously described [22] . The optimal (saturating) concentration of each GST-VP8* was initially determined from its dose-dependent cell-binding curve. For A-Tri blockade studies, A-Tri (2 mM or 10 mM final conc.) or DMEM was reacted for 1 H at 4 °C with the optimal level of GST-VP8* for HAL1166 (150 μg ml −1 ), K8 (600 μg ml −1 ) or Wa (300 μg ml −1 ), then added to cells for 45 min. Stained single cells were analysed by flow cytometry as previously described [22] . The results provided are representative of those obtained in three independent experiments. Assays for inhibition of rotavirus infectivity A-tri (2, 5 or 10 mM), H type-1 antigen (10 mM), Lewis b antigen (10 mM), rotavirus-neutralizing monoclonal antibody (as mouse ascites fluid) or DMEM diluent were incubated with trypsin-activated rotavirus for 1 h at 37 °C. The antibodies used were directed either to VP4 or to rotavirus outer capsid protein VP7, which confers glycoprotein (G) serotype specificity. Antibodies comprises the G8-specific B37:1 (ref. 63 ) (dilution: 1 in 1,000) for HAL1166, the G1-reactive RV-4:3 (ref. 64 ) (1 in 2,000) for K8, the G1-reactive IA10 (ref. 65 ) (1 in 10,000) for Wa, the G3-specific RV-3:1 (ref. 57 ) (1 in 20,000) for RV-3, the ST-3- and P[6]-specific ST-3:3 (ref. 66 ) (1 in 50,000) for ST-3 and the P[4]-specific RV-5:2 (ref. 67 ) (1 in 20,000) for DS-1. Confluent MA104 cell monolayers containing 4 × 10 4 cells were washed before virus-ligand mixtures or DMEM were transferred onto cells and reacted for 1 h at 37 °C at the optimum multiplicity of infection of 0.02. Following inoculum removal and washing as above, infected cells were incubated for 15 h at 37 °C in 95% (vol/vol) air with 5% (vol/vol) CO 2 . Acetone-fixed cell monolayers were sequentially stained with rabbit antiserum to rotavirus (1 in 1,000) and fluorescein isothiocyanate-conjugated goat anti-rabbit IgG (Invitrogen; 1 in 80), and virus titres determined by fluorescence microscopy as described previously [68] . For all assays, data represent the mean of triplicate samples and two independent experiments. Statistical analysis Student’s t -test was used, with significance set at the 95% level. Error bars on graphs indicate the s.d. How to cite this article: Böhm, R. et al . Revisiting the role of histo-blood group antigens in rotavirus host-cell invasion. Nat. Commun. 6:5907 doi: 10.1038/ncomms6907 (2015).